Mass production of two-dimensional oxides by rapid heating of hydrous chlorides Two-dimensional (2D) nanoscale oxides have attracted research interest owing to their electronic, magnetic optical and catalytic properties. If they could be manufactured on a large scale, 2D oxides would be attractive for applications ranging from electronics to energy conversion and storage. Herein, we report facile fabrication of oxide nanosheets by rapid thermal annealing of corresponding hydrous-chloride compounds. By heating CrCl 3 ·6H 2 O, ZrOCl 2 ·8H 2 O, AlCl 3 ·6H 2 O and YCl 3 ·6H 2 O crystals as precursors, we immediately collect large quantities of ultrathin Cr 2 O 3 , ZrO 2 , Al 2 O 3 and Y 2 O 3 nanosheets, respectively. The formation of layered nanosheets relies on exfoliation driven by rapid evaporation of water and/or other gas molecules generated under annealing. Our route allows simple, efficient and inexpensive production of 2D oxides. As a demonstration, we evaluate Cr 2 O 3 nanosheets prepared by our method as anodes in lithium-ion batteries and find superior performance in comparison with their microcrystalline counterparts. Materials of small geometrical dimensions have been successfully used in many technological applications because of their size-dependent physical and chemical properties [1] , [2] , [3] , [4] . In particular, the remarkable properties of graphene have renewed interest in inorganic two-dimensional (2D) materials with unique electronic, mechanical and optical attributes [5] , [6] , [7] , [8] , [9] , [10] . Beyond graphene, other 2D materials, such as transition metal dichalcogenides (for example, MoS 2 and WS 2 ), graphene analogues (for example, boron nitride), black phosphorus and some transition metal oxides (TMOs) (for example, MnO 2 and TiO 2 ) have attracted great attention because of their important applications in sensors, electrochemical catalysts and battery electrodes [11] , [12] , [13] , [14] , [15] , [16] , [17] , [18] . Scientists have reported multiple methods of preparing 2D nanosheets. One of the most common strategies used to prepare 2D nanolayers is mechanical or chemical exfoliation; some layered materials, such as BN, MoS 2 , MoSe 2 , MoTe 2 and TaSe, which have strong in-plane chemical bonds and weak out-of-plane van der Waals interactions, are easily exfoliated normal to the in-plane direction under extreme conditions [17] , [19] , [20] . A family of 2D nanosheets, labelled MXene, was produced through selective etching of the A-group atoms from MAX-phase solids such as Ti 3 AlC 2 (refs 21 , 22 , 23 , 24 ). Numerous 2D metal oxide nanosheets of materials such as TiO 2 , ZnO and MnO 2 can be fabricated by self-assembly or other wet chemistry methods [16] , [25] . Some nanosheets without layered crystal structures can also be synthesized from starting materials such as metals. For example, researchers have prepared ultrathin metal nanosheets from materials such as rhodium and gold via solvothermal and wet chemistry methods, respectively [26] , [27] . Although researchers have studied many methods to synthesize 2D materials, these methods are usually complex, expensive and inefficient. The lack of chemical or physical approaches to synthesizing ultrathin nanosheets in large quantities has limited further development and applications of these 2D materials. Therefore, a simple, fast and economical method for the mass production of 2D nanomaterials remains an interesting challenge [28] . In the liquid exfoliation method, ions or molecules are usually intercalated between layers to weaken the out-of-plane van der Waals interactions before the layer-structured materials are exfoliated [29] , [30] , [31] , [32] . Some layer-structured minerals with molecules between the layers also exist in nature, such as vermiculite. Vermiculite comprises a group of 2:1 phyllosilicate clay minerals that consist of hydrated sheet silicates that contain layers of water molecules within their internal structure [33] , [34] . When subjected to heat, vermiculite has the unusual property of expanding (commercial varieties can expand 8–20 times or more) because of the interlaminar generation of steam [33] , [34] . Accordingly, exfoliation of thin vermiculite layers occurs when the mineral is heated sufficiently ( Supplementary Fig. 1 ). Herein, inspired by the expansion and exfoliation that occur on heating of vermiculite, we apply rapid annealing to hydrous chlorides and oxychlorides and observe similar, large volume expansions. Using this approach, we successfully obtain sheets of layered oxides, including Cr 2 O 3 , ZrO 2 , Al 2 O 3 and Y 2 O 3 . The thinnest of the exfoliated oxide layers was ∼ 1.2 nm thick ( Supplementary Fig. 2 ) and spans several micrometres. Importantly, oxide nanosheets can be generated in large quantities by this rapid process. As a demonstration, Cr 2 O 3 synthesized by our technique was evaluated as an anode material in the Li-ion batteries. The 2D structure provides a larger and more stable surface area than do microparticles, enhancing capacities accessible at useful rates. Moreover, Cr 2 O 3 nanosheets show strong adhesion to the copper foil, even without binder, which enhances mechanical stability of electrodes during cycling. Materials design and synthesis Some metal oxide solids cannot be synthesized by direct exfoliation methods because they do not have layered crystal structures. However, some chlorides or oxychlorides of the corresponding metal oxides possess layered structures. In addition, the chlorides and oxychlorides usually have water in the crystal lattice, such as CrCl 3 ·6H 2 O, ZrOCl 2 ·8H 2 O, AlCl 3 ·6H 2 O and YCl 3 ·6H 2 O. When the hydrous chlorides or oxychlorides are heated under dry conditions or/and at high temperatures, the following four chemical reactions occur: During the dehydration and hydrolysis reactions in the rapid thermal process, a large quantity of gaseous reaction products, such as H 2 O and HCl, are produced within a short time, generating large pressures. The forces caused by gas evolution can drive exfoliation of layered solid products such as MCl x . The produced layers can further react spontaneously to form M 2 O x nanosheets ( Fig. 1a ). Accordingly, we are able to obtain 2D metal oxide nanosheets from hydrated precursors via a rapid thermal process. 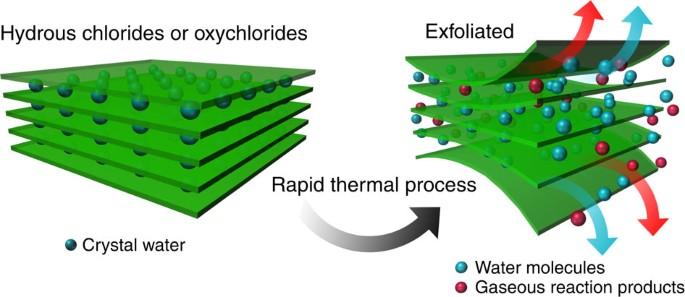Figure 1: Material synthesis. Schematic of the exfoliation of hydrous chlorides. During heating, large quantities of gas (water or other gaseous reaction products) are released. The force generated by gas generation and expansion leads to the exfoliation of the hydrates. Figure 1: Material synthesis. Schematic of the exfoliation of hydrous chlorides. During heating, large quantities of gas (water or other gaseous reaction products) are released. The force generated by gas generation and expansion leads to the exfoliation of the hydrates. Full size image Microwave heating is a common method used to heat or dry materials. The energy of the microwaves can be absorbed by water in a process called dielectric heating [35] , which is rapid and uniform. Accordingly, we used microwave heating to treat the CrCl 3 ·6H 2 O precursor. The morphology of the CrCl 3 ·6H 2 O particles is shown in a scanning electron microscopy (SEM) image ( Supplementary Fig. 3 ); the particles were not layered nanosheets. The CrCl 3 ·6H 2 O was placed in a glass bottle and then heated in a domestic microwave oven for 5 min. After heating, water was observed inside the bottle cap. The CrCl 3 ·6H 2 O in the glass bottle underwent a very large volume expansion ( Fig. 2a and Supplementary Movie 1 ). These observed phenomena were consistent with our expectations. The material obtained from CrCl 3 ·6H 2 O through microwave heating is deliquescent and must be stored under dry conditions. We used SEM and transmission electron microscopy (TEM) to examine the sample ( Fig. 2b,c ). Typical 2D nanosheets with relatively large areas were observed. The diffraction pattern ( Fig. 2c ) indicated that the sample was amorphous. We used energy-dispersive spectroscopy (EDS) to detect the chemical elements in the sample. The resulting atomic ratio for Cr, O and Cl of 1:1:1 suggested that the sample was CrOCl ( Supplementary Fig. 4a ). The reason that we did not obtain Cr 2 O 3 was likely insufficient heating power of the household microwave oven, leading to partial Cl removal. Although we collected CrOCl nanosheets using microwave heating, we investigated other rapid heating methods that could be used to obtain the oxides from CrCl 3 ·6H 2 O. 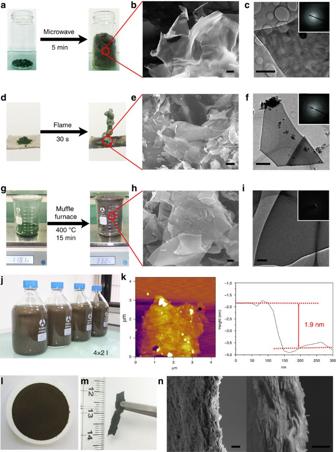Figure 2: Nanosheets produced from chromium trichloride hexahydrate. (a) A CrCl3·6H2O sample before (left of panel) and after (right of panel) microwave heating. (b) SEM and (c) TEM images (inset, corresponding electron diffraction pattern) correspond to the sample ina. (d) A CrCl3·6H2O sample before (left of panel) and after (right of panel) flame heating. (e) SEM and (f) TEM images (inset, corresponding electron diffraction pattern) correspond to the sample ind. (g) A CrCl3·6H2O sample before (left of panel) and after (right of panel) being heated in the muffle furnace. (h) SEM and (i) TEM images (inset, corresponding electron diffraction pattern) correspond to the CrCl3·6H2O sample ing. (j) A large quantity (8 l) of the 2D Cr2O3dispersion solution. (k) AFM characterization of the Cr2O3obtained by alcohol lamp heating. (l) The 2D Cr2O3film produced by vacuum filtration. (m) The free-standing 2D Cr2O3film. (n) Cross-sectional SEM images of the free-standing 2D Cr2O3film. Scale bars, 2 μm (b,c), 5 μm (e), 500 nm (f,i) and 10 μm (h,n). Figure 2: Nanosheets produced from chromium trichloride hexahydrate. ( a ) A CrCl 3 ·6H 2 O sample before (left of panel) and after (right of panel) microwave heating. ( b ) SEM and ( c ) TEM images (inset, corresponding electron diffraction pattern) correspond to the sample in a . ( d ) A CrCl 3 ·6H 2 O sample before (left of panel) and after (right of panel) flame heating. ( e ) SEM and ( f ) TEM images (inset, corresponding electron diffraction pattern) correspond to the sample in d . ( g ) A CrCl 3 ·6H 2 O sample before (left of panel) and after (right of panel) being heated in the muffle furnace. ( h ) SEM and ( i ) TEM images (inset, corresponding electron diffraction pattern) correspond to the CrCl 3 ·6H 2 O sample in g . ( j ) A large quantity (8 l) of the 2D Cr 2 O 3 dispersion solution. ( k ) AFM characterization of the Cr 2 O 3 obtained by alcohol lamp heating. ( l ) The 2D Cr 2 O 3 film produced by vacuum filtration. ( m ) The free-standing 2D Cr 2 O 3 film. ( n ) Cross-sectional SEM images of the free-standing 2D Cr 2 O 3 film. Scale bars, 2 μm ( b , c ), 5 μm ( e ), 500 nm ( f , i ) and 10 μm ( h , n ). Full size image The most immediate heating method is using a flame. The flame of an alcohol lamp is a dry environment and a high temperature ( ∼ 500 °C). We placed CrCl 3 ·6H 2 O crystals on nickel foam and heated the crystals in the flame of an alcohol lamp for 30 s. We again observed marked volume expansion ( Fig. 2d ). Most of the obtained sample was insoluble in water. Typical 2D nanosheets with large area were observed by SEM ( Fig. 2e ) and TEM characterization ( Fig. 2f ). The nanosheets were amorphous according to the diffraction pattern ( Fig. 2f ) and the high-resolution TEM (HRTEM) image ( Supplementary Fig. 5a ). EDS analysis ( Supplementary Fig. 5b ) indicated that the nanosheets were mainly composed of Cr and O, but Cl was also present. On the basis of the EDS and X-ray photoelectron spectroscopy (XPS) results ( Supplementary Fig. 5c ), we posited that the obtained nanosheets were amorphous chromium oxide. However, it is difficult to distinguish between Cr 2 O 3 and CrO 2 using XPS results. Although we believe that a portion of the Cr in the nonstoichiometric amorphous product is high-valence Cr, for convenience, we refer to the materials as amorphous Cr 2 O 3 . The thickness of the Cr 2 O 3 nanosheets was measured by atomic force microscopy (AFM). The thickness of the amorphous Cr 2 O 3 obtained by alcohol lamp heating reached 1.9 nm ( Fig. 2k ). However, we also observed some sheets that were composed of small crystalline particles ( Supplementary Fig. 5d,e ). In addition, the X-ray diffraction pattern also suggested that the sample contained crystallographic Cr 2 O 3 ( Supplementary Fig. 5f ). This result may be a consequence of the temperature distribution of the alcohol lamp flame being inhomogeneous, resulting in uneven heating of the CrCl 3 ·6H 2 O crystals, which caused the sample to be non-uniform. We therefore changed the heating method from flame heating to a more homogeneous heating method to obtain uniform amorphous Cr 2 O 3 nanosheets. A muffle furnace can control temperature and maintain it at a constant level. This heating method is more homogeneous and capable of treating more samples. We set the temperature of the muffle furnace at 400 °C. The CrCl 3 ·6H 2 O crystals were placed in a quartz crucible, directly placed into the furnace at 400 °C and treated for 15 min. After the heating process, the raw CrCl 3 ·6H 2 O material exhibited large volume expansion ( Fig. 2g and Supplementary Movie 2 ). Most of the obtained sample was insoluble in water, and large-area layered materials were observed by optical microscopy ( Supplementary Fig. 6a ). We observed a large quantity of 2D sheets by SEM ( Fig. 2h ). In addition, according to the diffraction pattern ( Fig. 2i ) and HRTEM results ( Supplementary Fig. 6b ), the nanosheets were amorphous. The EDS ( Supplementary Fig. 6c ) and XPS analysis results ( Supplementary Fig. 6d ) showed the samples mainly consisted of Cr and O with a small amount of Cl; the results also indicated that the obtained material was amorphous Cr 2 O 3 nanosheets. Compared with the density of normal Cr 2 O 3 ( ∼ 5.21 g ml −1 ), the tap density of the expanded Cr 2 O 3 was very low, ∼ 0.0332, g ml −1 . Using this method, we could mass-produce Cr 2 O 3 nanosheets as shown in Supplementary Fig. 7a . For instance, we could fabricate 1,000 ml of Cr 2 O 3 nanosheets in ∼ 2 h in the lab using only a small muffle furnace (the interior dimensions of the furnace are ∼ 10 × 10 × 10 cm 3 , as shown in Supplementary Fig. 7b ). After removing the soluble impurities, the production yield of the Cr 2 O 3 nanosheets is around 88%. We could also prepare 8 l of an aqueous Cr 2 O 3 nanosheet solution at a concentration of 3 g l −1 ( Fig. 2j ). The Cr 2 O 3 solution could be used to prepare free-standing films of Cr 2 O 3 by vacuum filtration ( Fig. 2l,m ). Figure 2n shows a cross-section of the free-standing Cr 2 O 3 films. Such solution-based methods are favourable for practical applications such as preparing and processing electrode slurries. In addition to the rapid heating treatment, we also annealed CrCl 3 ·6H 2 O crystals under a gradually increasing temperature profile; samples were heated from room temperature to 400 °C at 5 °C min −1 in a muffle furnace and maintained at 400 °C for 15 min. We observed the expected volume expansion, but we did not observe predominant quantities of smooth, large-area nanosheets. Most of the resulting sample was in the form of thick sheets formed by small particles ( Supplementary Fig. 8 ). This result suggests that the hydrous chloride crystals could be exfoliated and further reacted to form oxides by heat treatment. However, layer thickness may be influenced by the rate of temperature increase; the exfoliated oxide sheets gradually crystallize to form small Cr 2 O 3 crystal particles during the slow heat-treatment process. Accordingly, the rate of temperature increase during the heating treatment is key to obtaining ultrathin 2D metal oxide nanosheets. Electrochemical performance of the Cr 2 O 3 nanosheets To explore the application of our exfoliated 2D Cr 2 O 3 nanosheets, we incorporated the amorphous Cr 2 O 3 nanosheets into Li-ion batteries. Lithium can be stored reversibly in TMOs through the following reaction: Among TMOs, Cr 2 O 3 is suitable as an anode material for Li-ion batteries because of its high theoretical capacity (1,058 mAh g −1 ), low average charging voltage ( ∼ 1.2 V) and low electromotive force value (1.085 V versus Li/Li + ) [36] , [37] . However, the cycling performance of Cr 2 O 3 electrodes is poor because of a loss of electronic contact of active materials and poor electron and ion transport properties within the active material [36] . We investigated whether use of our 2D Cr 2 O 3 nanosheets as active materials could address these limitations. We fabricated graphene/2D Cr 2 O 3 composite electrodes. The graphene and Cr 2 O 3 were assembled layer by layer because of their similar 2D layered structure. The stacked 2D structure can provide good electrical contact between the graphene and Cr 2 O 3 nanosheets, improving electron transport. The ultrathin, 2D layered structure can help access to the active material by the electrolyte and aid ion transport. We fabricated graphene/Cr 2 O 3 (2D) electrodes and graphene/Cr 2 O 3 (particle)/polyvinylidene difluoride (PVDF) electrodes, as mentioned in the Methods section. The cells were tested over a voltage range from 0 to 3 V versus Li + /Li. During the test, the initial lithiation and delithiation capacity of the graphene/Cr 2 O 3 (particle)/PVDF electrodes was only ∼ 738 and 316 mAh g −1 , respectively, and the delithiation capacity decreased to only 168 mAh g −1 after ∼ 10 cycles at the current density of 0.2 A g −1 ( Fig. 3a ). By contrast, the graphene/Cr 2 O 3 (2D) electrodes exhibited a high capacity and stable cycling performance. The graphene/Cr 2 O 3 (2D) electrodes achieved an initial delithiation capacity of 974 mAh g −1 at a rate of 0.2 A g −1 . After 297 cycles, the capacity was ∼ 986 mAh g −1 , and the cell continued to function well ( Fig. 3a ). This electrochemical performance of the graphene/Cr 2 O 3 (2D) electrodes is excellent compared with the reported performance of other Cr 2 O 3 electrodes [38] , [39] , [40] , [41] , [42] . The galvanostatic lithiation/delithiation profiles and rate performance of our 2D Cr 2 O 3 electrodes are included in Fig. 3b,c . We measured the impedance of the electrodes by electrochemical impedance spectroscopy in terms of Nyquist plots ( Supplementary Fig. 9 ). The semicircle in high-frequency region is related to the solid electrolyte interphase (SEI) film and the medium-frequency semicircle due to the charge transfer resistance, and the inclined line in the low-frequency region represents the diffusion of lithium ions [43] , [44] . The surface film resistance, which originates from the SEI, and the charge transfer resistance of the graphene/Cr 2 O 3 (particle)/PVDF electrode were 12.3 and 56.9 Ω, respectively. However, the graphene/Cr 2 O 3 (2D) composites showed lower SEI and charge transfer resistances, which were 6.6 and 21.4 Ω. The electrochemical impedance spectroscopy results indicated the interface of graphene/Cr 2 O 3 (2D) electrodes is more stable and confirmed the 2D structure is attributed to the charge transfer and charge diffusion, which could support the good electrochemical and rate performances of graphene/Cr 2 O 3 (2D) electrodes. Importantly, the graphene/Cr 2 O 3 (2D) composites exhibited strong adhesion to the current collector (copper foil) and between the layers. The graphene/Cr 2 O 3 (2D) electrodes and graphene/Cr 2 O 3 (particle)/PVDF electrodes were immersed in the electrolyte solution; we then sonicated the electrodes in the electrolyte solution with ultrasonic cleaning (80 W, 40 kHz) for 5 min. For the graphene/Cr 2 O 3 (particle)/PVDF electrodes, the PVDF binder did not prevent the spalling of the electrode material from the current collector during the ultrasonic cleaning process ( Fig. 3e ). However, the graphene/Cr 2 O 3 (2D) composite materials remained on the current collector ( Fig. 3d ). We also tested the adhesion of the two electrode types by cleaning them ultrasonically in water and ethyl alcohol. The graphene/Cr 2 O 3 (2D) electrodes maintained structural stability in all three solutions, whereas the graphene/Cr 2 O 3 (particle)/PVDF electrodes exhibited different degrees of spalling ( Supplementary Fig. 10 ). We used the scotch tape method to mechanically remove material from the electrodes. While the graphene/Cr 2 O 3 (particle)/PVDF electrode was easily peeled off, the graphene/Cr 2 O 3 (2D) electrodes remained intact and no stripping happened ( Fig. 3f and Supplementary Movie 3 ). The observed strong adhesion and the structural stability of our graphene/2D Cr 2 O 3 composite materials could explain the stable electrochemical performance of the graphene/Cr 2 O 3 (2D) electrodes. We suggest the strong adhesion has three potential causes. First, the 2D structure of Cr 2 O 3 provides a high contact area with graphene and copper foil, and the calendaring process ensures good contact between Cr 2 O 3 (2D), graphene and copper foil. Second, according to zeta potential measurements under neutral conditions, graphene was negatively charged (−9.26 mV) and the 2D Cr 2 O 3 was positively charged (32.5 mV), suggesting that electrostatic attraction contributes to the adhesion between 2D Cr 2 O 3 and graphene. Third, and finally, we speculate that some chemical bonding may occur at the interface between the electrode material and current collector, between amorphous Cr 2 O 3 nanosheets and the copper foil due to the high-valence Cr and low-coordinated surface atoms, leading to robust adhesion to the copper foil [45] , [46] . Such adhesion properties are interesting for applications in many fields, such as flexible energy storage devices or chemical coatings. 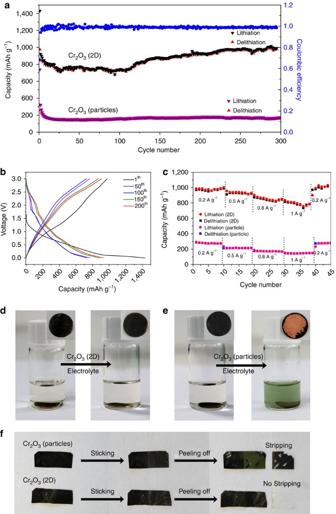Figure 3: Electrochemical and adhesion performance of chromic oxides. (a) The cycling performance of the Cr2O3electrodes. (b) The galvanostatic lithiation/delithiation profiles of the 2D Cr2O3electrodes. (c) The rate performance of the Cr2O3electrodes. (d) The Cr2O3(2D) electrode and (e) Cr2O3(particles) electrode before (left of panel) and after (right of panel) being ultrasonically cleaned in an electrolyte solution. (f) The Cr2O3electrodes before and after mechanical exfoliation. Figure 3: Electrochemical and adhesion performance of chromic oxides. ( a ) The cycling performance of the Cr 2 O 3 electrodes. ( b ) The galvanostatic lithiation/delithiation profiles of the 2D Cr 2 O 3 electrodes. ( c ) The rate performance of the Cr 2 O 3 electrodes. ( d ) The Cr 2 O 3 (2D) electrode and ( e ) Cr 2 O 3 (particles) electrode before (left of panel) and after (right of panel) being ultrasonically cleaned in an electrolyte solution. ( f ) The Cr 2 O 3 electrodes before and after mechanical exfoliation. Full size image Extended material systems Beyond the chromium oxides from the CrCl 3 ·6H 2 O, we applied the rapid heating method to other hydrous chlorides to obtain metal oxides such as ZrO 2 , Al 2 O 3 and Y 2 O 3 . The ZrOCl 2 ·8H 2 O, AlCl 3 ·6H 2 O and YCl 3 ·6H 2 O crystals were not layered nanosheets before the rapid heating treatment ( Supplementary Fig. 11 ). The ZrOCl 2 ·8H 2 O starting material was heated in the microwave oven for 10 min. A portion of the obtained sample dissolved in water, and we collected the insoluble portion. Typical nanosheets were obtained, as shown by optical microscopy ( Supplementary Fig. 12a ), SEM ( Fig. 4a ) and TEM images ( Fig. 4b ). On the basis of the EDS ( Supplementary Fig. 12c ) and XPS ( Supplementary Fig. 12d ) results, we deduced the nanosheets to be ZrO 2 . The diffraction pattern ( Fig. 4b ) and HRTEM results ( Supplementary Fig. 12b ) indicated that the 2D ZrO 2 sheets were amorphous. 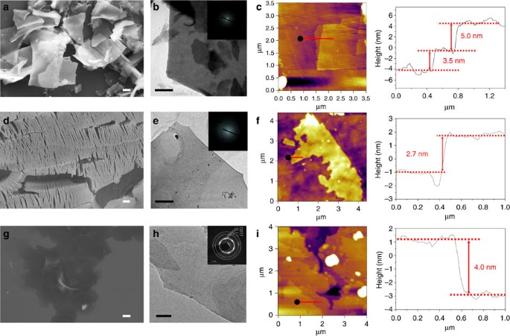Figure 4: Characterizations of the oxide nanosheets. (a) SEM, (b) TEM (inset, corresponding electron diffraction pattern) and (c) AFM characterizations of the ZrO2nanosheets. (d) SEM, (e) TEM (inset, corresponding electron diffraction pattern) and (f) AFM characterizations of the Al2O3nanosheets. (g) SEM, (h) TEM (inset, corresponding electron diffraction pattern) and (i) AFM characterizations of the Y2O3nanosheets. Scale bars, 2 μm (a,d,g), 500 nm (b,e) and 50 nm (h). Figure 4: Characterizations of the oxide nanosheets. ( a ) SEM, ( b ) TEM (inset, corresponding electron diffraction pattern) and ( c ) AFM characterizations of the ZrO 2 nanosheets. ( d ) SEM, ( e ) TEM (inset, corresponding electron diffraction pattern) and ( f ) AFM characterizations of the Al 2 O 3 nanosheets. ( g ) SEM, ( h ) TEM (inset, corresponding electron diffraction pattern) and ( i ) AFM characterizations of the Y 2 O 3 nanosheets. Scale bars, 2 μm ( a , d , g ), 500 nm ( b , e ) and 50 nm ( h ). Full size image In the case of the AlCl 3 ·6H 2 O crystals, we placed the crystals in a glass bottle and heated them for ∼ 5 min using the alcohol lamp. After the heat treatment, the exfoliated sample was observed by SEM ( Supplementary Fig. 13 ), although inidividual sheets were difficult to distinguish. We therefore chose an alternative method to produce Al 2 O 3 sheets. We used a heating gun to generate hot air with a maximum temperature of ∼ 500 °C. We prepared an AlCl 3 solution (1 g ml −1 ) in water and painted the solution onto copper foil. The copper foil was then dried in an oven at 60 °C for ∼ 30 min to obtain a hydrous AlCl 3 thin film. We heated the hydrous AlCl 3 on the copper foil using the heating gun ( ∼ 500 °C) until the light-yellow solid appeared. We observed that the solid formed on the copper foil was exfoliated Al 2 O 3 ( Fig. 4d ); ultrathin nanosheets were observed using TEM ( Fig. 4e ). These sheets were amorphous Al 2 O 3 according to the diffraction pattern ( Fig. 4e ), HRTEM, EDS and XPS results ( Supplementary Fig. 14 ). We also produced Y 2 O 3 nanosheets using the rapid heat-treatment furnace, which could heat to hundreds of degrees within a few seconds. The heating principle of the rapid heat treatment furnace is light radiation, and the process generates strong air flow. The light radiation heats the hydrous chlorides and causes water and hydrogen chloride molecules to escape from the crystals. The air flow removes the water and hydrogen chloride molecules from the environment, which favours the escape of more gas molecules. We treated YCl 3 ·6H 2 O samples in this furnace. The YCl 3 ·6H 2 O was placed in a crucible, heated to 600 °C, and maintained at this temperature for 2 min in the rapid heat-treatment furnace. Although the samples were not uniform and contained numerous particles, we still obtained Y 2 O 3 nanosheets, as indicated by SEM, TEM ( Fig. 4g,h ) and EDS results ( Supplementary Fig. 15b ). The diffraction pattern ( Fig. 4h ) and HRTEM ( Supplementary Fig. 15a ) results indicated that part of the Y 2 O 3 nanosheets was crystallized (PDF#44–0399), but the crystallinity was poor. We measured the thickness of the metal oxide nanosheets using AFM. The thinnest layers of the ZrO 2 , Al 2 O 3 and Y 2 O 3 obtained by rapid heating methods exhibited layer thicknesses of 3.5, 2.7 and 4.0 nm, respectively ( Fig. 4c,f,i ). We could collect the 2D nanosheets using different combinations of the aforementioned materials and heating methods. For example, we obtained amorphous Cr 2 O 3 nanosheets by heating the CrCl 3 ·6H 2 O in the rapid heat treatment furnace ( Supplementary Fig. 16 ). Some precursors without crystal water (such as anhydrous AlCl 3 ) or without layered crystal structure (such as AlNO 3 ·9H 2 O) were also treated by the rapid heating process, however the 2D oxides were not obtained in these cases ( Supplementary Figs 17 and 18 ), which strengthens our point about the formation mechanism of oxide nanosheets. Although we obtained metal oxides using the various methods previously mentioned, the idea of treating the hydrous chloride with a rapid thermal process is consistent. The differences are the heating principles and specific procedures. However, the influential factors and manufacturing techniques require further improvement and study because the products obtained were not uniform and because we could not produce other TMOs to the same degree as we could produce the Cr 2 O 3 nanosheets. We produced the 2D Cr 2 O 3 nanosheets on a large scale within a short time (that is, several minutes) by rapidly heating hydrous chlorides; the 2D Cr 2 O 3 showed excellent electrochemical performance in Li-ion battery and surprisingly strong adhesion to the copper foil substrate. We also demonstrated that this method of producing ultrathin nanosheets could be generalized to allow rapid production of other oxides such as ZrO 2 , Al 2 O 3 and Y 2 O 3 . We believe that this concept provides a practically promising avenue for simple, efficient, fast and inexpensive production of large quantities of large-area, ultrathin 2D nanosheets. Synthesis of 2D CrOCl by microwave heating The CrCl 3 ·6H 2 O crystals were placed in a glass bottle and heated using a microwave oven for ∼ 5 min. Then, the obtained CrOCl materials were transferred and stored in an Ar-filled glove box. The CrOCl nanosheets were dispersed in benzene to prepare TEM samples. Synthesis of the 2D oxides The CrCl 3 ·6H 2 O crystals were placed on nickel foam and heated using an alcohol lamp for ∼ 2 min; or placed in a quartz crucible and heated in a muffle furnace at 400 °C for ∼ 15 min. The ZrOCl 2 ·8H 2 O crystals were placed in a glass bottle and heated using a microwave oven for ∼ 10 min. The AlCl 3 ·6H 2 O crystals were dissolved in deionized water at a concentration of 1 g ml −1 , and the solution was painted onto copper foil. The copper foil was dried in an oven at 60 °C for 30 min to obtain the hydrous AlCl 3 thin film. We heated the hydrous AlCl 3 on the copper foil using a heating gun until a white or light-yellow solid appeared. The white or light-yellow solid was Al 2 O 3 nanosheets. The YCl 3 ·6H 2 O crystals were placed in an alumina crucible and heated in the rapid heat treatment furnace at 600 °C for ∼ 2 min. The obtained metal oxide products contain incompletely reacted intermediate products. We dispersed the obtained products in deionized water to remove the soluble impurities. The dispersion of products was centrifuged for 5 min at 12,000 r.p.m. to obtain the sediment. We repeated the centrifuging process three times to clean the products (the first two times using deionized water and the third time using ethyl alcohol). The obtained sediment was dried in an oven at 80 °C. Battery electrodes based on nanosheets or on microparticles We dispersed graphene (10 wt%) and Cr 2 O 3 nanosheets (90 wt%) in water at a concentration of 10 mg ml −1 (total mass). We also dispersed graphene (10 wt%), Cr 2 O 3 particles ( ∼ 300 nm, 80 wt%) and PVDF (10 wt%) in N-methyl-2-pyrrolidone (NMP) at a concentration of 10 mg ml −1 (total mass). The composite slurry was dropped onto a flat copper foil and dried in an oven at ∼ 80 °C. The dried electrodes were pressed using a calendaring process ( ∼ 20 MPa). The mass loading of the electrodes was ∼ 0.5 mg cm −2 . The electrodes were assembled into half-cells with Li metal foil (MTI) as a counter electrode in an Ar-filled glove box. We used a 25 μm-thick microporous polypropylene membrane as the separator (Asahi Kasei) and 1 M LiPF 6 in ethylene carbonate/diethyl carbonate/fluoroethylene carbonate (1:1:0.04 vol/vol/vol, Ferro Corporation) as the electrolyte. Characterization The X-ray diffraction patterns of the rare materials and products were evaluated using a D/max-2500 diffractometer (Rigaku, Japan) equipped with a CuK α radiation source. The chemical states of the products were determined by XPS (Thermo Fisher ESCALAB 250Xi). The morphology of the samples was observed with a SEM (MERLIN VP Compact, ZEISS, Germany). The chemical composition of the samples was analysed using EDS (X-Max N , Oxford Instruments). HRTEM observation was carried out using JEOL-2100 TEM operated at 200 kV. The thickness of the nanosheets was determined by AFM (MFP-3D, Asylum Research, Oxford Instruments). The electrochemical performances of the batteries were measured by a BS-9300R/10V2A MTI 8 channels battery analyser. Data availability The data that support the findings of this study are available from the corresponding author on request. How to cite this article: Zhao, C. et al . Mass production of two-dimensional oxides by rapid heating of hydrous chlorides. Nat. Commun. 7:12543 doi: 10.1038/ncomms12543 (2016).